Biophysical mechanisms that maintain biodiversity through trade-offs Trade-offs are thought to arise from inevitable, biophysical limitations that prevent organisms from optimizing multiple traits simultaneously. A leading explanation for biodiversity maintenance is a theory that if the shape, or geometry, of a trade-off is right, then multiple species can coexist. Testing this theory, however, is difficult as trait data is usually too noisy to discern shape, or trade-offs necessary for the theory are not observed in vivo . To address this, we infer geometry directly from the biophysical mechanisms that cause trade-offs, deriving the geometry of two by studying nutrient uptake and metabolic properties common to all living cells. To test for their presence in vivo we isolated Escherichia coli mutants that vary in a nutrient transporter, LamB, and found evidence for both trade-offs. Consistent with data, population genetics models incorporating the trade-offs successfully predict the co-maintenance of three distinct genetic lineages, demonstrating that trade-off geometry can be deduced from fundamental principles of living cells and used to predict stable genetic polymorphisms. Trade-offs between life-history traits are seen as a key part of the processes that maintain the rich biodiversity observed in microbes [1] , plants [2] , insects [3] and rain forests [4] . Due to its importance to biodiversity theory, a search for trade-off data has become the subject of a burgeoning experimental literature using microbial populations in the laboratory [1] , [5] , [6] , [7] , [8] , [9] , [10] , [11] , [12] . However, despite the significance of trade-off geometry to the theory and the long-postulated hypothesis that trade-offs arise from life-history constraints, we know of no successful derivation of trade-off geometry in living systems from fundamental physical or biochemical principles. Resolving this absence is critical if we are to successfuly predict conditions that maintain diverse microbial communities. Here we present a mechanistic theory, supported by data, on the geometry of two trade-offs among microbes: one is a feeding trade-off, one is a growth trade-off. These trade-offs have been studied before but their shapes have remained elusive, yet here we find agreement between theory and data showing that one trade-off is convex and the other is sigmoidal and both are implicated in diversity maintenance. The first trade-off we study is the metabolic rate–yield trade-off (the RYTO or ‘waste from haste’ trade-off [13] , [14] ) whose shape we found by culturing Escherichia coli at different growth rates. The second trade-off shape we deduce is that of the nutrient uptake rate-affinity trade-off (the RATO [14] , [15] ) by measuring the growth kinetics of a library of mutant E. coli that varied in a sugar transporter, LamB. Given these two geometries, prior theory predicts that there could be nutrient conditions where divergent consumer strategies would coexist in a microbial population [16] . To test this, we used bespoke theoretical population genetics models to determine environmental conditions that would support a multiplicity of nutrient transporter genotypes in E. coli . However, this theory successfully predicted the frequency dynamics of three genetic lineages in a laboratory microcosm only when it incorporated two trade-offs, not one. We therefore establish that trade-offs are a consequence of the physical necessities of life and moreover genetic polymorphisms and biodiversity patterns can be predicted from the resulting trade-off geometries. Many mechanisms have been proposed for the RYTO in bacteria, both physiological [17] and metabolic [13] , and a quadratic shape is thought to describe it [13] . Attempts to find the RYTO in vivo , however, have been mixed. A negative correlation between growth rate and yield has been observed but without the quadratic form [12] . Moreover, positive rate–yield correlations, the antithesis of a rate–yield trade-off, have been observed in other bacterial species [9] and, curiously, this relationship is also predicted to be constrained by a quadratic geometry [10] . We can reconcile these apparent contradictions by following a suggestion [9] that r – k relationships can be manipulated by varying the carbon richness of the environment in which bacteria grow (for clarity, we use k for carrying capacity where others use K ). We hypothesize that r and k are indeed positively correlated and that the shape of the RYTO can be extracted from r–k data sets. To study the RYTO, we cultured E. coli B (REL606) in Davis minimal (DM) medium supplemented with a range of sugar (maltotriose) concentrations. We determined their r (exponential growth rate) and k (maximal population size) values by fitting the mathematical logistic model to growth data, where x ( t ) denotes bacterial population density at time t ( Supplementary Discussion , section C). At low sugar concentrations, ranging from 1 to 8 μg ml −1 the experiment recapitulates a prior data set [9] , whereby a positive, linear correlation between r and k is observed ( Fig. 1a ). However, when observations from higher maltotriose concentrations are added to the data, ranging from 1 to 125 μg ml −1 , the r–k relationship becomes nonlinear because r saturates. This is expected because growth rate is limited, whereas k increases proportionally to the maltotriose supplied ( Fig. 1a , Supplementary Fig. 15 ). Although r and k adaptation are classically viewed as conflicting life-history strategies [18] here they are positively correlated. Nevertheless, this is still consistent with a RYTO, as we now explain. 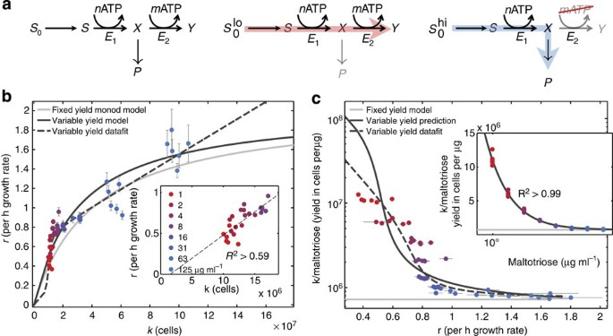Figure 1: The RYTO shape can be derived from a simple branched metabolic pathway model and subsequently found in bacterial growth data. (a) A branched pathway predicts that cell yield,c, can be written in the form of equation (1) (derivation inSupplementary Discussion, section B). (b) AsS0increases to 125 μg ml−1,rbegins to saturate, whereaskcontinues to increase. Moreover, two theoretical Monod models (light and dark grey) assuming, respectively, fixed and variable yield are both compatible with this (k,r) data set. (binset) WhenS0ranges from 1 to 8 μg ml−1,randkappear linearly correlated, an observation consistent with published data9(error bars indicate mean±s.e.m., horizontal s.e.m. bars are present but cannot be seen, six replicates per maltotriose concentration). (c) The variable-yield model (Equation 2) was used to estimate rate–yield trade-off geometry: the solid line shows the predicted geometry using the data set from (b), the dashed line improves on this prediction by fitting equation (2) directly to that data set (Supplementary Table 2contains relevant parameter estimates). Both of these trade-off models are sigmoidal, note, and the resulting predicted growth rate is shown as a dashed line inb. (cinset) A constant yield assumption fails when yield is plotted versus maltotriose concentration (light grey line). The nonlinear yield form from equation (1),c(S0), correctly captures the data (dark grey line). Figure 1: The RYTO shape can be derived from a simple branched metabolic pathway model and subsequently found in bacterial growth data. ( a ) A branched pathway predicts that cell yield, c , can be written in the form of equation (1) (derivation in Supplementary Discussion , section B). ( b ) As S 0 increases to 125 μg ml −1 , r begins to saturate, whereas k continues to increase. Moreover, two theoretical Monod models (light and dark grey) assuming, respectively, fixed and variable yield are both compatible with this ( k , r ) data set. ( b inset) When S 0 ranges from 1 to 8 μg ml −1 , r and k appear linearly correlated, an observation consistent with published data [9] (error bars indicate mean±s.e.m., horizontal s.e.m. bars are present but cannot be seen, six replicates per maltotriose concentration). 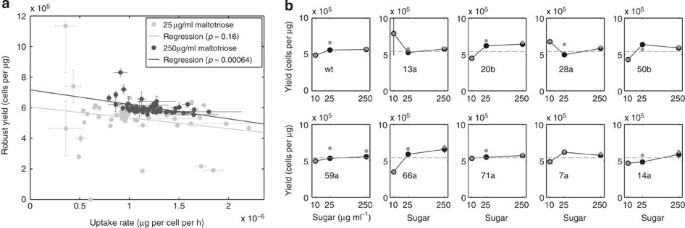Figure 2: The evidence for a between-strain RYTO is not significant at all maltotriose concentrations tested. (a) Estimated maltotriose uptake rate versus a robust estimate of cell yield (Supplementary Discussion, section C) for every genotype in thelamBmutant library at two different maltotriose supply concentrations (S0=25 and 250 μg ml−1). Linear regressions show evidence of a between-strain negative correlation in yield but only whenS0=250 (error bars indicate mean±s.d.,n=8; regression:R2≈0.21,F-statistic versus constant model: 13.3,P<0.00064). (b) Ten strains from the library exhibit a feature common to all: although there are fluctuations due to experimental variation, cell yield is estimated consistently between strains across a range of maltotriose concentrations (error bars indicate mean±s.e.m.,n=3; black and grey dots represent two different yield estimation algorithms, the horizontal dashed line is mean wild-type yield). ( c ) The variable-yield model (Equation 2) was used to estimate rate–yield trade-off geometry: the solid line shows the predicted geometry using the data set from ( b ), the dashed line improves on this prediction by fitting equation (2) directly to that data set ( Supplementary Table 2 contains relevant parameter estimates). Both of these trade-off models are sigmoidal, note, and the resulting predicted growth rate is shown as a dashed line in b . ( c inset) A constant yield assumption fails when yield is plotted versus maltotriose concentration (light grey line). The nonlinear yield form from equation (1), c ( S 0 ), correctly captures the data (dark grey line). Full size image Assume, for the moment, that c is a constant representing the biomass yield of E. coli per maltotriose, when cultured with maltotriose as the sole carbon source at supply concentration S 0 μg ml −1 . We assume Monod growth kinetics, so the bacterial population density B changes as and maltotriose reduces in concentration as , where V max is the maximal rate of uptake of maltotriose and K m is the maltotriose half saturation constant. The initial condition S (0)= S 0 applies here, B (0) represents a bacterial inoculate whose size is assumed negligibly small. A conservation law holds in this model, B ( t )/c+ S ( t )= B (0)/c+ S 0 , so that when S ≈0 at carrying capacity, k = B ≈c· S 0 thus k is proportional to the maltoriose supplied, if we neglect B (0). If we approximate exponential growth using the Monod model, so r ≈c V max S 0 /( K m + S 0 ), then k / r ≈( K m + S 0 )/ V max and so k and k / r should both exhibit linear dependence on S 0 , hence k and r should be positively correlated. This is consistent with our observations (for k versus S 0 : R 2 >0.99, P <10 −8 ; for k / r versus S 0 : R 2 ≈0.93, P <10 −4 ; Supplementary Fig. 15 ). However, observations also indicate that yield, meaning c or k / S 0 , is not constant because it decreases with increasing maltotriose supply ( Fig. 1b , F -test versus constant model, F =17.3, P <0.00014). We therefore need a more accurate description of the variable-yield data in Fig. 1c . So, we relax our assumption that yield is a constant independent of the carbon supplied. Maltotriose import and metabolism is carried out by the genes of the mal regulon [19] . This set is induced by malT , which itself is expressed when maltodextrins like maltotriose are present. The uptake of maltodextrins is facilitated by the LamB maltoporin in combination with the periplasmic maltodextrin-binding protein MalE and the ATP-driven inner-membrane transport system MalGFK 2 . Once in the cytoplasm, maltotriose is degraded by MalZ into maltose and glucose, MalQ then produces two glucoses for each available maltose. Given this, a theoretical form for the rate and yield of maltose metabolism can be derived ( Supplementary Discussion , section B) by representing glycolysis and the tricarboxylic acid (TCA) cycle as a branched pathway [20] ( Fig. 1a ). Using ATP yield as a proxy for biomass yield, this model predicts a relationship between carbon supply, S 0 , and cell yield. Writing c ( S 0 ) to represent this relationship, it has the following repression-activation form Here c hi represents the highest yield attainable, achieved at the lowest sugar concentrations, whereas c lo is the yield attained when sugar is abundant, p is a phenotype that controls the rate of decrease in yield with increasing sugar supply. The positive r–k correlation predicted by the constant and variable-yield assumptions are consistent with r–k data ( Fig. 1b ) with agreement across 2 orders of magnitude of maltotriose supply in both cases. However, only the decreasing yield model correctly captures the yield data across the full range of maltotriose concentrations ( Fig. 1c , R 2 >0.99, P ≪ 10 −15 from above F -test). The resulting five-parameter, within-strain geometric RYTO model has a sigmoidal shape that compares favourably with data ( Fig. 1c ). Note that equation (2) has only four independent parameters, V max merely converts cell yield into a rate. The logistic equation contains no explicit term for nutrient availability so, we deployed the following improvement to that model that better captures different bacterial growth phases and which can also represent N -strain, frequency- and density-dependent competition for maltotriose (where N ≥1): Here B i is density of the i -th strain, growth rate is G i ( S )= c i · U i ( S ), c i is cell yield and U i ( S ) is nutrient uptake rate (at nutrient concentration S ): The variable n i represents a subpopulation of the inoculate that may be in a non-vegetative state and the associated ν i -dependent terms allow the model to capture the transition from lag to exponential phase. When N =1 equation (3) is consistent with the RYTO data for E. coli strain REL606 ( Supplementary Fig. 14 ) and when N >1, it can predict the outcome of multi-strain competition experiments ( Supplementary Discussion , section C). Pursuing evidence of a between-strain RYTO, we generated a library of E. coli mutants that vary in growth rate because of mutations that interfere with maltotriose uptake. E. coli uses LamB to transport maltotriose across the outer membrane, however, it may also be taken up by OmpF, albeit over an order of magnitude more slowly [21] , [22] . LamB is also a receptor for the virus λ, which provides a convent way to generate LamB mutations. Previous work has shown that when E. coli and λ are co-cultured, E. coli rapidly evolves resistance through an array of lamB mutations [23] , [24] , some of which alter the diffusion of maltodextrins across the outer membrane by altering the pore dimensions [25] . We therefore co-cultured 100 separate populations in batch for 3 days and isolated 2 bacteria per population. The large number of populations and low sampling intensity within each population helped maximize the number of unique lamB mutants isolated, the short time period ensured only a single mutation occurred in the lamB gene and nowhere else in the genome. Altogether, we harvested 50 novel E. coli strains with SNPs, insertions and deletions in the lamB gene, the library also includes frameshift mutations that render LamB inoperable ( Supplementary Table 1 ). We estimated uptake rate, yield and therefore growth rate for each strain by culturing them separately in DM media supplemented with 10, 25 and 250 μg ml −1 maltotriose by fitting equation (3) to that data ( Supplementary Discussion , section C). This consistently produced similar values for yield between strains and environments and significant evidence for a negative rate–yield correlation between strains was observed but only at a maltotriose concentration of 250 μg ml −1 , not at 25 μg ml −1 ( P <0.00064 and P >0.16, respectively; see Fig. 2a ). Figure 2: The evidence for a between-strain RYTO is not significant at all maltotriose concentrations tested. ( a ) Estimated maltotriose uptake rate versus a robust estimate of cell yield ( Supplementary Discussion , section C) for every genotype in the lamB mutant library at two different maltotriose supply concentrations ( S 0 =25 and 250 μg ml −1 ). Linear regressions show evidence of a between-strain negative correlation in yield but only when S 0 =250 (error bars indicate mean±s.d., n =8; regression: R 2 ≈0.21, F -statistic versus constant model: 13.3, P <0.00064). ( b ) Ten strains from the library exhibit a feature common to all: although there are fluctuations due to experimental variation, cell yield is estimated consistently between strains across a range of maltotriose concentrations (error bars indicate mean±s.e.m., n =3; black and grey dots represent two different yield estimation algorithms, the horizontal dashed line is mean wild-type yield). Full size image The same data set points to a second possible trade-off: a correlation between K m and V max ( Fig. 3a , R 2 ≈0.58, F ≈70.5, P <10 −10 ). This prediction is consistent with prior single transporter models for small-molecule uptake, which show that changes to a transporter’s affinity for the molecule will produce concomitant changes in its maximal translocation rate [26] , [27] , [28] . This was demonstrated by distorting the performance of transmembrane channels by creating potential energy wells within a synthetic pore using holographic tweezers. These experiments showed that an optimal transporter configuration must balance a high translocation probability and ‘not too long’ a blockage of the channel [27] ; this is the physical basis of the RATO. 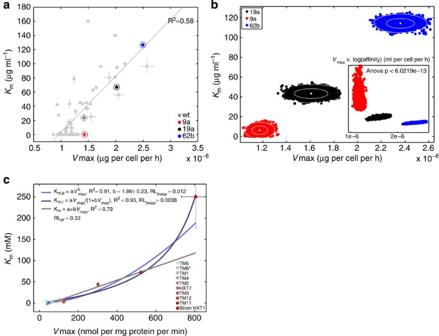Figure 3: RATO data in theE. colilibrary is too noisy to discern a nonlinear shape, however, a priorSaccharomyces cerevisiaedata set has a nonlinear RATO. (a) An indication that theE. colilibrary is consistent with a between-strain RATO: estimated values ofKmandVmaxare positively correlated (error bars indicate mean±s.e.m.,n=8). (b) Maximum likelihood estimates of (Km,Vmax) for library strains 9a, 19a and 62b showing ~70 and 95% confidence contours of marginal posterior distributions determined using the Matlab MCMC Toolbox (MLEs ofKm: 0.011 mM, 0.080 mM and 0.211 mM, respectively. As a comparison,E. colistrains from the literature38have values ~0.4 mM). (binset) Using this data, library strains were isolated (9a, 19a and 62b) that exhibit a between-strain RATO (see analysis of variance in main text). (c) A whole cellS. cerevisiae(Km,Vmax) data set (mean data and standard error bars from ref.26) exhibits a nonlinear uptake RATO. Two robust geometric data fits are shown next to the robust linear regressionKm=a+bVmax: a near-quadratic power law,Km,pand a rational functionKm,r. Relative likelihoods of the two nonlinear fits indicate both are significantly better descriptors of the data than a linear function (the indicated RLlinearvalues are the relative likelihoods for each fit). This demonstrates consistency between the predicted nonlinear RATO shape (equation 5) and data. Figure 3: RATO data in the E. coli library is too noisy to discern a nonlinear shape, however, a prior Saccharomyces cerevisiae data set has a nonlinear RATO. ( a ) An indication that the E. coli library is consistent with a between-strain RATO: estimated values of K m and V max are positively correlated (error bars indicate mean±s.e.m., n =8). ( b ) Maximum likelihood estimates of ( K m , V max ) for library strains 9a, 19a and 62b showing ~70 and 95% confidence contours of marginal posterior distributions determined using the Matlab MCMC Toolbox (MLEs of K m : 0.011 mM, 0.080 mM and 0.211 mM, respectively. As a comparison, E. coli strains from the literature [38] have values ~0.4 mM). ( b inset) Using this data, library strains were isolated (9a, 19a and 62b) that exhibit a between-strain RATO (see analysis of variance in main text). ( c ) A whole cell S. cerevisiae ( K m , V max ) data set (mean data and standard error bars from ref. 26 ) exhibits a nonlinear uptake RATO. Two robust geometric data fits are shown next to the robust linear regression K m = a + bV max : a near-quadratic power law, K m,p and a rational function K m,r . Relative likelihoods of the two nonlinear fits indicate both are significantly better descriptors of the data than a linear function (the indicated RL linear values are the relative likelihoods for each fit). This demonstrates consistency between the predicted nonlinear RATO shape (equation 5) and data. Full size image Different theories are possible for RATO geometries depending on the assumptions they use. A linear relationship between K m and V max can be derived [27] (as is done in equation (6) of the latter reference), whereby K m = pV max + q for parameters ( p , q ). This result is consistent with a theoretical enzymatic model based on a transporter embedded within a single membrane ( Supplementary Discussion , section B), so this would appear to be the description of the trade-off we seek. However, affinity for a carbon source, a , is usually defined by and so strains with different V max and K m phenotypes could have a common maltotriose affinity, if q =0. However, RATO data observed between the E. coli library strains is too noisy to eliminate linearity or to resolve shape ( Fig. 3a ). To remedy this, we used a related Saccharomyces cerevisiae data set where glucose transporters had been genetically manipulated [26] . As this data exhibits significant nonlinearity (see Fig. 3b for the relative likelihoods, RL linear , of linear and nonlinear data fits where RL linear <0.013), the prior argument supporting a linear K m – V max relationship will thus have to be modified. On reflection, small-molecule uptake in some microbes is a two-step process: entry into the cytoplasm of Gram-negative bacteria and yeast requires the passage through two diffusive barriers, not one. Modifying the above single membrane model to account for this, K m depends nonlinearly on V max in the resulting theory ( Supplementary Discussion , section B): where ( p , q , r , s ) are parameters. A quadratic nonlinearity here is expected because if transport through one diffusive barrier leads to a linear K m – V max relationship, two barriers positioned in serial separated by a periplasm should produce a quadratic-like function, which equation (5) is. A power-law fit to empirical ( V max , K m ) data of the form is consistent with equation (5) because b ≈1.86±0.23 (mean±estimated s.e.m., degree of freedom=8, Fig. 3b ). We note that the role played by MalE in E. coli is neglected as part of the derivation of equation (5) (in Supplementary Discussion , section B), but if we were to assume that MalE–maltotriose binding is so rapid that no free maltotriose is found in the periplasm, then the form of equation (5) will not change. To test whether the RATO could promote the maintenance of bacterial diversity, we isolated a subset of our library that exhibited a RATO. Three strains, labelled 9a (a predicted high-affinity strain; an AAC deletion at 871 bp in lamB ), 19a (a frameshift mutant with nonfunctional LamB, T insertion at 610 bp) and 62b (predicted low-affinity strain; A→G at 1,211 bp) were identified with different maltotriose transport properties ( Fig. 3b ), one-way analysis of variance, F ≈28.2, P <7 × 10 −13 ). The three-strain version of equation (3) predicts they should coexist in a fluctuating resource environment, such as a batch culture, where bacteria are inoculated into fresh flasks each day with high initial resources that are depleted throughout a 24-h cycle as the bacteria grow ( Fig. 4a ). 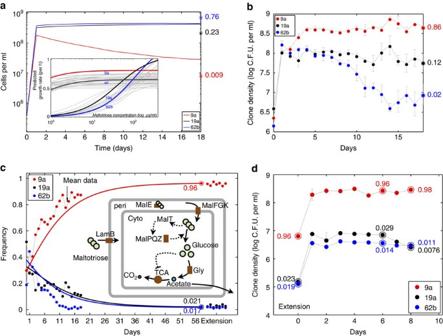Figure 4: As predicted by population genetics theory, threelamBmutant strains can be stably co-maintained in a laboratory microcosm. (a) A theoretical three-strain co-culture model (N=3 in a seasonal extension of equation 3) containing a RATO but no RYTO predicts strain dynamics for 18 days when maltotriose is supplied each day at 300 μg ml−1. Maltotriose uptake rates, affinities and yields were estimated for each strain in monoculture and the inset shows estimated growth rate for every library strain: strains 9a, 19a and 62b are predicted to have fastest growth in different maltotriose concentration windows. (b) While the model correctly predicts the co-maintenance of three strains, this was not at the strain frequencies that were subsequently observed. Note, 62b has mean population size on day 18 of over one million cells (colony-forming units) despite a mean relative frequency of 2.4% (error bars indicate mean±s.e.m.,n=3). (c) A RYTO was then introduced into the model that was used to make the predictions inaand the resulting model is consistent with strain frequencies (Supplementary Discussion, section D). One model simulation is shown (thick lines) superimposed on observed mean strain frequencies (dots). (cinset) The internal complexity of theE. colistrains on which simulations incare based, assuming only polymorphisms inlamB. (d) The three strains were co-cultured anew in the same conditions but this time they were inoculated at the model-predicted steady state frequencies, these frequencies were then maintained for a period of 7 days (Supplementary Discussion, section D). Mean observed frequencies are shown next to the model predictions incby the label ‘extension’, the observed densities of this extension are shown ind. Note: numerical text labels in each plot indicate relative frequencies of each strain. Figure 4: As predicted by population genetics theory, three lamB mutant strains can be stably co-maintained in a laboratory microcosm. ( a ) A theoretical three-strain co-culture model ( N =3 in a seasonal extension of equation 3) containing a RATO but no RYTO predicts strain dynamics for 18 days when maltotriose is supplied each day at 300 μg ml −1 . Maltotriose uptake rates, affinities and yields were estimated for each strain in monoculture and the inset shows estimated growth rate for every library strain: strains 9a, 19a and 62b are predicted to have fastest growth in different maltotriose concentration windows. ( b ) While the model correctly predicts the co-maintenance of three strains, this was not at the strain frequencies that were subsequently observed. Note, 62b has mean population size on day 18 of over one million cells (colony-forming units) despite a mean relative frequency of 2.4% (error bars indicate mean±s.e.m., n =3). ( c ) A RYTO was then introduced into the model that was used to make the predictions in a and the resulting model is consistent with strain frequencies ( Supplementary Discussion , section D). One model simulation is shown (thick lines) superimposed on observed mean strain frequencies (dots). ( c inset) The internal complexity of the E. coli strains on which simulations in c are based, assuming only polymorphisms in lamB . ( d ) The three strains were co-cultured anew in the same conditions but this time they were inoculated at the model-predicted steady state frequencies, these frequencies were then maintained for a period of 7 days ( Supplementary Discussion , section D). Mean observed frequencies are shown next to the model predictions in c by the label ‘extension’, the observed densities of this extension are shown in d . Note: numerical text labels in each plot indicate relative frequencies of each strain. Full size image We cultured 9a, 19a and 62b in DM with 300 μg ml −1 of maltotriose for 18 days in such a batch culture microcosm and found that, consistent with predictions, all three genotypes persisted. However, the model is not quantitative ( Fig. 4b ): it fails to predict the relative frequencies at which each genotype was maintained. Most notably, the microcosm was dominated by the high-affinity strain, 9a, whereas the model predicts that the low-affinity strain, 62b, should prevail ( Fig. 4a ). This shows that consumer lifestyle and the between-strain RATO alone are not sufficient to explain the dynamics we observe. To understand why theory and experiments disagreed, we reasoned that the RYTO could play a role because it could lead fast-uptake genotypes to have low efficiencies which would impact growth rates. To justify this we followed the path of maltotriose through the cell which is converted to glucose and an excess of glucose produced at high maltotriose concentrations will lead glycolytic NADH to repress citrate synthase and, therefore, the TCA cycle [29] . As total ATP yield from the TCA cycle is greater per glucose supplied than from glycolysis, this repression should strengthen the within-strain RYTO we observed ( Fig. 1 ). We therefore included a glucose-dependent, maltotriose-to-biomass conversion efficiency into the model to mimic the RYTO ( Supplementary Discussion , section D). Only then, with two trade-offs, do we have a theory consistent with the 18-day mean frequency dynamics of the strains that also exhibits the long-term coexistence of all three ( Fig. 4c ). To test for stable coexistence, we inoculated the three strains into a fresh microcosm at relative frequencies predicted by the trained dual trade-off model after running it to equilibrium. After so doing, we found no evidence of a deviation from the predicted strain frequencies when propagating them for further 7 days of seasonal co-culture ( Fig. 4c and Supplementary Discussion , section D). The eventual deviation that we observed of the microcosm from the theoretical prediction is only to be expected as the coexisting lineages likely gain further mutations that are not encoded within the model ( Supplementary Discussion , section D). Trade-off shape is believed to be a key to understanding species diversity in global ecosystems and our analyses concur. Our theoretical models and empirical analyses elucidate the shape of two, the RATO and RYTO. According to our theory, both must be invoked simultaneously to explain the stable maintenance of genetic diversity in an E. coli transporter gene, lamB , when mutants are co-cultured within a seasonal resource dynamic. The RATO, with its quadratic shape ( Fig. 3b ), is the result of a biophysical constraint that arises because the transport of extracellular nutrients into the cell is optimized. As different transporter structures are optimal for different extracellular nutrient concentrations, a continuum of potential sugar uptake niches is created ( Fig. 4a ) that here maintains three genetic lineages. However, nutrient consumption alone cannot account for strain frequencies and differential efficiencies resulting from downstream metabolism due to the RYTO, with its sigmoidal shape ( Fig. 1c ), ensure that efficient and not greedy consumers prevail. Trade-offs have long been postulated as a mechanism supporting genetic diversity in ecosystems and it has become a fundamental problem in ecology to find them in living systems [30] . Importantly, we show they are predictable: because trade-offs are the result of physical processes within the cell, their shapes can be derived mathematically and corroborated against empirical data. Consistent with trade-off theories of biodiversity, we also show that polymorphisms in specific feeding genes are predictable. However, just one trade-off was not enough, we need to account for the simultaneous presence of two to correctly predict allele frequencies in a bacterial microcosm. Therefore, theories of multiple simultaneous trade-offs [31] are likely needed to capture the diversity observed in natural ecosystems. lamB mutant library generation We co-cultured E. coli strain B(REL606), from the laboratory of Richard Lenski, Michigan State University, Michigan, USA, with the obligatorily lytic λ strain cI26, from the laboratory of Donald Court, National Cancer Institute, Maryland, USA. When co-cultured with cI26, REL606 experiences strong pressure to evolve resistance because E. coli B strains lack generalized phage defenses such as mucoid cell formation, restriction modification or CRISPR adaptive immunity [32] , [33] . This pressure is magnified by the lytic phage’s increased virulence as compared with its lysogenic relatives [34] . About 100 flasks were initiated with 10 3 bacterial cells and even fewer phage (~10 2 particles). We initiated the study with small populations to increase the likelihood that mutations for defense would arise de novo , which improved our chances of isolating unique lamB mutations. Culturing occurred in 50 ml Erlenmeyer flasks, filled with 10 ml of modified DM [35] (125 μg ml −1 maltotriose instead of glucose and 1 μg ml −1 of magnesium sulphate), incubated for 24 h, at 37 °C and shaken at 120 r.p.m. Bacteria were pre-conditioned for a full 24-h cycle before being co-cultured with phage. After the first 24 h of incubation in the mixed cultures, a random 100 μl sample of each flask was transferred to a fresh flask and the bacteria and phage were allowed to grow again. This cycle was repeated twice and bacteria were sampled after the third day of growth. We ended the experiment at this early time-point to ensure that the bacteria only had enough time to evolve a single mutation for defense. In addition, in previous experiments we observed the greatest genotypic diversity of bacteria on the third day. E. coli evolve resistance in this environment through mutations in many loci, however, preliminary experiments revealed that lamB is the most common locus for λ resistance mutations. For this study, we focused just on genotypes that had mutations in lamB . Bacterial isolation and storage To isolate bacteria we streaked a sample on Luria Bertani (LB) agar plates [36] , incubated them for 24 h at 37 °C, and arbitrarily picked two colonies. Next, we re-plated each colony two more times serially to remove all phage. Finally, we grew each colony in liquid LB overnight and preserved two 1 ml samples in 15% glycerol and froze it at −80 °C. We tested whether each isolate had evolved resistance to λ by spot assay [37] , where 2 μl of the concentrated phage stock is dried on top of a matrix of 4 ml of soft agar (LB agar with only 4% w/v agar) and 0.5 ml of the LB overnight culture. The matrix is suspended on top of a typical LB agar Petri dish. Each plate was incubated at 37 °C for 24 h and then scored the next day. A strain was considered resistant if no clearing occurred under the spot where the phage lysate was applied. We sequenced each of the resistant genotypes to determine if resistance had evolved through mutations in lamB . Sequencing Sequencing was performed with an automated ABI sequencer maintained at Michigan State University Research Technology Support Facility. PCR-amplified fragments that were purified with GFX columns and were used as templates. Fragments containing lamB were amplified with primer sequences 5′-TTCCCGGTAATGTGGAGATGC-3′ and 5′-AATGTTTGCCGGGACGCTGTA-3′, placed 1,398 bases up and 504 bases downstream of the lamB gene, respectively. Growth dynamics Each genotype was revived by inoculating a few microliters of frozen culture into a tube with 4 ml of liquid LB. Cultures were grown at 37 °C and shaken at 160 r.p.m. After 12 h, 10 μl of each culture was transferred to a fresh tube with modified DM250 and grown for 12 h at 37 °C and shaken at 160 r.p.m. This acclimation step to DM250 was repeated again because preliminary studies showed that growth was much more consistent when two sequential acclimation steps were performed. Finally, 2 μl of each culture (10 6 cells) was inoculated into a well with 200 μl of modified DM. Wells were randomized in a 96-well plate, however, cultures were never inoculated into the outer-rim to avoid edge effects caused by increased rates of evaporation. Next, the cells were incubated at 37 °C and the optical densities (at 420 nm wave length) of each well was measured once every 5 min for 12 h using a VersaMax automated plate reader (Molecular Devices). Each genotype was grown in modified DM supplemented with either 25 μg ml −1 of maltotriose or 250 μg ml −1 , in four separate replicates. Optical densities (OD) was converted into cell densities by comparing counts of colony-forming units to ODs at a number of different cell concentrations. Growth curves were created identically for the ancestor, REL606, except at many more concentrations of maltotriose (1, 2, 4, 8, 16, 32, 64 and 128 μg ml −1 ). These data were used to measure the RYTO. Coexistence experiments Coexistence experiments were run under the same conditions as the growth dynamics were measured, except maltotriose concentrations were increased to 333 μg ml −1 , plates were continuously shaken at 220 r.p.m. and the experiments were run for 18 days by transferring a random sample of 2% of the culture after 24 h of growth to a well with fresh medium. Coexistence was measured by tracking co-occurring populations of three genotypes—9a, 19a and 62b. To track the populations, we used the ara genetic marker. Each of the three lamB mutant genotypes were unable to metabolize L-arabinose ( ara- ) because of a single nucleotide substitution in araA that caused a G-to-D amino acid change at position 92. We selected for spontaneous reversions of this mutation by growing ~10 9 cells of each strain on minimal arabinose plates for 48 h at 37 °C (ref. 35 ). Reversions were verified by targeted sequencing of araA using the same protocol for lamB , except the following primers were used for PCR amplification: 5′-CCGATACGCTCATGGGCTTGTTTA-3′ and 5′-CTGCCCAGGCCGTTGCGACTCTAT-3′. The ara genetic marker was chosen because previous work has shown that it does not confer a cost [35] . We cultured each ara + genotype with the ara − version of the other two lamB mutants. The density of the focal genotype was measured by counting colonies on minimal arabinose plates. Total bacterial population size was also measured by counting colonies on LB plates. For each ara + genotype, we constructed four replicate populations making 12 coexistence experiments in total. How to cite this article : Meyer, J. R. et al . Biophysical mechanisms that maintain biodiversity through trade-offs. Nat. Commun. 6:6278 doi: 10.1038/ncomms7278 (2015).